FtsZ-independent septal recruitment and function of cell wall remodelling enzymes in chlamydial pathogens The nature and assembly of the chlamydial division septum is poorly defined due to the paucity of a detectable peptidoglycan (PG)-based cell wall, the inhibition of constriction by penicillin and the presence of coding sequences for cell wall precursor and remodelling enzymes in the reduced chlamydial (pan-)genome. Here we show that the chlamydial amidase (AmiA) is active and remodels PG in Escherichia coli . Moreover, forward genetics using an E. coli amidase mutant as entry point reveals that the chlamydial LysM-domain protein NlpD is active in an E. coli reporter strain for PG endopeptidase activity (Δ nlpI) . Immunolocalization unveils NlpD as the first septal (cell-wall-binding) protein in Chlamydiae and we show that its septal sequestration depends on prior cell wall synthesis. Since AmiA assembles into peripheral clusters, trimming of a PG-like polymer or precursors occurs throughout the chlamydial envelope, while NlpD targets PG-like peptide crosslinks at the chlamydial septum during constriction. The stress-bearing peptidoglycan (PG)-based cell wall protects bacterial cells from physical and chemical insults. PG (also known as murein) synthesis occurs throughout the envelope and at the division septum [1] , [2] . The septal PG along with constriction force by the cytokinetic ring assembled from FtsZ tubulin directs the envelope into an annular structure at the division plane to enable membrane fusion, ultimately compartmentalizing the dividing cell into two separate daughter chambers ( Fig. 1a ) [3] , [4] . The building block of PG is lipid II, an N -acetyl-glucosamine(GlcNAc)- N -acetyl-muramic acid (MurNAc)-pentapeptide unit carried by the phosphorylated isoprenoid bactoprenol (C55~\nP). During PG synthesis, the MurNAc-GlcNAc disaccharide units are polymerized into linear glycan strands by transglycosylase enzymes. The growing polymer is further fortified by crosslinking of the pentapeptide moieties by transpeptidases known as penicillin-binding proteins (PBPs; Fig. 1b ). Upon synthesis of the septal PG and the ensuing compartmentalization, the septal PG is split to accommodate daughter cell separation, a task executed by PG remodelling enzymes such as lytic transglycosylases, amidases ( N -acetylmuramoyl- L -alanine hydrolases) and peptidases (LD-carboxypeptidases and DD-endopeptidases) that act on the glycan, amide or peptide bonds in PG, respectively ( Fig. 1a,b ) [3] . 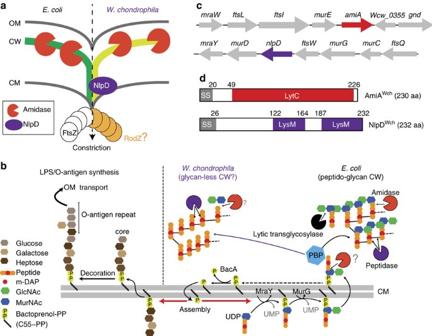Figure 1: Model of cell wall remodelling in dividingE. coliandW. chondrophila. (a) Coordinated envelope constriction inE. coliandW. chondrophila, a member of theChlamydialesorder, by the cytokinetic machinery and (putative) cell wall biosynthetic and remodelling enzymes including amidases and the putative endopeptidase NlpD fromW. chondrophila(NlpDWch). RodZWchwas recently identified as an early recruit to the division plane, raising the possibility that it acts in an early cytokinetic event11. (b) Schematic of cell wall assembly pathway inE. coliand the predicted pathway of a PG-like cell wall inW. chondrophila, as well as the O-antigen pathway for biosynthesis of LPS in theE. coliouter membrane (OM). Note that both pathways use bactoprenol (C55~\nP) as membrane carrier for precursor assembly. The possible removal of the dissaccharide unit from PG or lipid II is indicated with a question mark and a transparent dissaccharide unit. (c) Gene organization of the region encompassing the coding sequences for AmiA and NlpD inW. chondrophila. Arrows indicate gene orientation in theW. chondrophilagenome. (d) Predicted domain organization ofW. chondrophilaAmiA and NlpD. SS, signal sequence; LytC, (Pfam PF01520) amidase_3 domain; LysM, (Pfam PF01476) LysM-like PG-binding domain. Numbers refer to amino-acid positions in the translation product. Figure 1: Model of cell wall remodelling in dividing E. coli and W. chondrophila. ( a ) Coordinated envelope constriction in E. coli and W. chondrophila , a member of the Chlamydiales order, by the cytokinetic machinery and (putative) cell wall biosynthetic and remodelling enzymes including amidases and the putative endopeptidase NlpD from W. chondrophila (NlpD Wch ). RodZ Wch was recently identified as an early recruit to the division plane, raising the possibility that it acts in an early cytokinetic event [11] . ( b ) Schematic of cell wall assembly pathway in E. coli and the predicted pathway of a PG-like cell wall in W. chondrophila , as well as the O-antigen pathway for biosynthesis of LPS in the E. coli outer membrane (OM). Note that both pathways use bactoprenol (C55~\nP) as membrane carrier for precursor assembly. The possible removal of the dissaccharide unit from PG or lipid II is indicated with a question mark and a transparent dissaccharide unit. ( c ) Gene organization of the region encompassing the coding sequences for AmiA and NlpD in W. chondrophila . Arrows indicate gene orientation in the W. chondrophila genome. ( d ) Predicted domain organization of W. chondrophila AmiA and NlpD. SS, signal sequence; LytC, (Pfam PF01520) amidase_3 domain; LysM, (Pfam PF01476) LysM-like PG-binding domain. Numbers refer to amino-acid positions in the translation product. Full size image In addition to providing constriction force, FtsZ organizes septal PG synthesis and remodelling events [1] , [2] . Although most bacteria rely on FtsZ for division, several bacterial lineages, such as pathogens belonging to the phylum Chlamydiae , do not encode primary structural homologues of FtsZ in their genomes [1] . Thus, alternative organizers of PG synthesis/remodelling and of cytokinesis must exist. In principle, owing to their obligate intracellular life style and a protective network of proteins with disulphide bridges on the surface of elementary bodies (the infectious extracellular developmental stage), Chlamydiae should not need PG for protection from osmotic stress. Interestingly, however, despite the massive reduction in coding capacity of chlamydial genomes, a seemingly functional lipid II biosynthetic pathway along with several putative PG biosynthetic (transpeptidases, for example, FtsI) and predicted remodelling enzymes (putative amidases and endopeptidases) are encoded [5] , [6] , [7] , [8] . The latter suggests that chlamydial pathogens polymerize a septal PG derivative (or at least a PG remnant). Indeed, immunofluorescence labelling with antibodies to the Ribi adjuvant that contains mycobacterial cell wall skeleton or direct fluorescent labelling of a modified D -amino acid dipeptide revealed a non-proteinaceous PG-like substance or at least a dipeptide-derived PG precursor at the septum [9] , [10] . Moreover, penicillins (inhibitors of PBPs) block chlamydial division [8] , [10] , [11] . However, no coding sequences for known PG transglycosylation enzyme homologues are found in the genomes of chlamydial pathogens [8] , raising the intriguing possibility that this PG-like material lacks chains of glycan polymers and that instead the disaccharide units from lipid II remain unpolymerized after transpeptidation. Alternatively, unknown transglycosylation enzymes may promote glycan chain formation within the chlamydial cell wall. Modification of PG-like material, its synthesis in reduced amounts and/or its confinement in space or time could reflect an adaptation of chlamydial pathogens to the host by reducing the activation of NOD1/2 intracellular pattern recognition receptors that detect MurNAc-containing muropeptide fragments [12] . Division in the absence of classical PG and FtsZ as that seen for the L-form bacteria and mycoplasmas belonging to the phylum Firmicutes occurs in an erratic and inefficient manner by membrane blebbing, budding or stretching [1] , [13] , [14] . By contrast, cell division in the phylum Chlamydiae is highly coordinated and regular, resembling the binary fission of cocci [8] , [15] . It is unknown how chlamydia execute division and if they remodel their septal PG-like material, but recently the first septal proteins of Chlamydiae have been identified [11] . Escherichia coli mutants lacking all three amidase paralogues offer a convenient system to probe for septal PG remodelling by amidase-like activities, as inactivation of the three amidase genes ( amiA , amiB and amiC ) prevents cell separation, yielding a chaining phenotype [16] . Interestingly, the barrier function of the outer membrane (conferred by lipopolysaccharide [17] (LPS), which also uses C55~\nP as a carrier for the biosynthesis of its precursor; Fig. 1b ) is compromised in the Δ amiA , Δ amiB ; Δ amiC (henceforth Δ ABC ) triple mutant for reasons that are unclear [18] . Here, using E. coli Δ ABC as a surrogate host, we first confirmed that chlamydial AmiA orthologues restore cell separation and LPS barrier function, indicating that they are indeed active amidases. We then isolated a suppressive mutation in the E. coli gene encoding the NlpI lipoprotein that restores LPS function and alters the PG peptide crosslinking ratio in Δ ABC cells. We provide evidence that chlamydial NlpD can bind PG in vitro and that it has PG peptidase activity in E. coli cells that are mutant for nlpI in vivo . Importantly, immunolocalization of dividing chlamydial ( Waddlia chondrophila ) cells unveils NlpD as the first septal cell-wall-binding protein and shows that it depends on a PG-like polymer for localization to the division septum. As AmiA is distributed in the cell envelope, our results support a model in which AmiA trims a PG-like polymer or lipid II throughout the envelope, while NlpD acts on peptide crosslinks at the division septum of human chlamydial pathogens. Activity and peripheral localization of chlamydial amidases As chlamydial pathogens are typically small and difficult to grow, we exploited the robust growth and larger cell size of W . chondrophila , a member of the Chlamydiales order and a strict intracellular pathogen associated with bovine abortion and human miscarriage, for immunolocalization studies [19] , [20] . As it has so far not been possible to engineer targeted gene disruptions in W . chondrophila as for most members of the Chlamydiales , we complemented our cytological experiments with functional studies using E. coli as a surrogate host. W. chondrophila AmiA (AmiA Wch ) is encoded in a gene cluster with predicted cell division and PG precursor (lipid II) biosynthesis enzymes ( Fig. 1c ). Akin to other chlamydial AmiA orthologues, AmiA Wch exhibits 43% similarity (113/259) and 27% identity (70/259) to E. coli AmiA (AmiA Eco ), and features the predicted catalytic residues within the LytC/Amidase_3 signature domain of amidases ( Fig. 1d , Supplementary Fig. 1 and Supplementary Table 1 ). Interestingly, primary structure predictions suggest that chlamydial amidases lack the autoinhibitory alpha-helix ( Supplementary Fig. 1 ) that occludes substrate access of the E. coli amidases and that must first be displaced by a cognate amidase activator for the acquisition of full enzymatic activity [21] , [22] . This raises the possibility that the active site of the chlamydial amidase homologues could be in a constitutively open (active) state. AmiA Wch was able to rescue the cell separation defect (chaining phenotype) of the E. coli Δ ABC mutant ( Fig. 2a and Supplementary Fig. 2A ) akin to AmiA Eco . However, a significant amount of cell debris (‘ghosts’; arrowheads in Fig. 2a and Supplementary Fig. 2A ) accumulated in the cultures expressing AmiA Wch , presumably reflecting lysed cells from ectopic (un-restrained) amidase activity of AmiA Wch ( Fig. 2a ) that cannot be properly controlled by E. coli . In support of this, we observed by way of a LacZ-based lysis assay that AmiA Wch liberated LacZ much more efficiently from cells compared with AmiA Eco ( Supplementary Fig. 2B ). Cell ‘ghosts’ were not seen when AmiA Wch derivatives with single, double and/or quadruple mutations in key catalytic residues (H55A, E70A, H124A and/or E194A; Supplementary Fig. 1 ) or AmiA Eco were expressed ( Fig. 2a ), indicating that catalytic activity underlies the lysis phenotype. The catalytic mutants were also unable to support cell separation even though wild-type ( WT ) and most mutant AmiA Wch derivatives accumulated to comparable steady-state levels as determined by immunoblotting using polyclonal antibodies to AmiA Wch ( Supplementary Fig. 2C,D ). Finally, to determine whether these functional characteristics are also retained in AmiA orthologues from other members of the Chlamydiales , we conducted complementation experiments with a plasmid expressing the AmiA orthologue from Simkania negevensis (AmiA Sne ) or from Parachlamydia acanthamoebae (AmiA Pac ) [23] ( Supplementary Fig. 1 ) and found that both are also active as amidases, inducing lysis and supporting cell separation and ghost cell formation in E. coli ( Supplementary Figs 2B,E,F and 3A–C ). 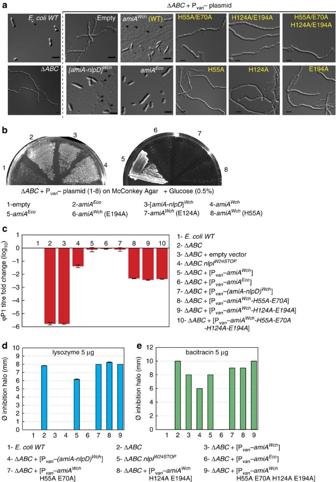Figure 2:W. chondrophilaAmiA supports cell separation inE. coliΔABCcells. (a) DIC images ofWTand ΔABC; ΔABC+Pvan-empty, -amiAWch, -[amiA-nlpD]Wchand -amiAEco. Arrowheads point to ghost cells; Scale bar, 4 μm. AmiA point mutants are highlighted in yellow. (b) Growth ofWTand mutantE. colistrains on McConkey agar supplemented with 0.5% glucose (McCG). (c) ϕP1 titre in the indicated strains were calculated as described in Methods and is reported as the log10fold change. Error bars show the s.d. Data are from three biological replicates. (d) Lysozyme sensitivity of the indicatedE. colistrains. 0.25 ml of saturated cultures were added to 5 ml of LB top agar and plated, the indicated amount of lysozyme was then spotted on the cell overlay and incubated overnight at 30 °C. Differences in sensitivity are reported as the difference in size (diameter) of the inhibition halo (mm). Error bars show the s.d. Data are from three biological replicates. (e) Bacitracin sensitivity of the indicatedE. colistrains. 250 microliters of saturated cultures were added to 5 ml of LB top agar and plated, the indicated amount of bacitracin was then spotted on the cell overlay and incubated overnight at 30 °C. Differences in sensitivity are reported as the difference in size (diameter) of the inhibition halo (mm). Error bars show the s.d. Figure 2: W. chondrophila AmiA supports cell separation in E. coli Δ ABC cells. ( a ) DIC images of WT and Δ ABC ; Δ ABC+ P van -empty, - amiA Wch , -[ amiA-nlpD ] Wch and - amiA Eco . Arrowheads point to ghost cells; Scale bar, 4 μm. AmiA point mutants are highlighted in yellow. ( b ) Growth of WT and mutant E. coli strains on McConkey agar supplemented with 0.5% glucose (McCG). ( c ) ϕP1 titre in the indicated strains were calculated as described in Methods and is reported as the log 10 fold change. Error bars show the s.d. Data are from three biological replicates. ( d ) Lysozyme sensitivity of the indicated E. coli strains. 0.25 ml of saturated cultures were added to 5 ml of LB top agar and plated, the indicated amount of lysozyme was then spotted on the cell overlay and incubated overnight at 30 °C. Differences in sensitivity are reported as the difference in size (diameter) of the inhibition halo (mm). Error bars show the s.d. Data are from three biological replicates. ( e ) Bacitracin sensitivity of the indicated E. coli strains. 250 microliters of saturated cultures were added to 5 ml of LB top agar and plated, the indicated amount of bacitracin was then spotted on the cell overlay and incubated overnight at 30 °C. Differences in sensitivity are reported as the difference in size (diameter) of the inhibition halo (mm). Error bars show the s.d. Full size image Further evidence that the chlamydial amidases indeed have lytic activity came from expression of WT and mutant AmiA Wch in the Gram-negative Alpha-proteobacterium Caulobacter crescentus that naturally grows in hypo-osmotic fresh water niches [24] and is thus more prone to lysis when PG integrity is compromised. We observed that WT AmiA Wch , but not mutant derivatives, induced rapid lysis upon shifting aerated (shaking) C . crescentus cultures to stasis ( Fig. 3a ). Moreover, high-performance liquid chromatography (HPLC) analysis of muropeptides liberated from purified cell wall sacculi that had been digested with the N -acetyl-muramidase mutanolysin revealed that AmiA Wch induces the appearance of several muropeptide fragments in C. crescentus that are not present in the control samples (from cells harbouring the empty vector), with a commensurate reduction in other muropeptide species ( Fig. 3b ). 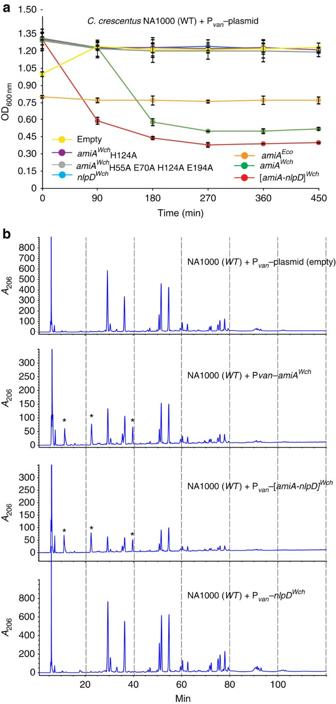Figure 3: Effect of AmiAWchderivatives on lysis ofCaulobacter crescentus. (a) Overnight cultures ofC. crescentusharbouring different constructs were left static at 30 °C and OD600 nmwere recorded every 90 min. Lysis occurred in strains carrying [Pvan−amiAWch] and [Pvan−(amiA-nlpD)Wch] while OD600 nmof strains carrying [Pvan−amiAWchH124A], [Pvan−amiAWchH55A E70A H124A E194A], [Pvan−nlpDWch] and pMT335 were not affected. Error bars show the s.d. Data are from three biological replicates. (b) Muropeptide analysis ofCaulobacter crescentuscell walls in the indicated strains harbouring different constructs as indicated on the figure. Differences among HPLC profiles are highlighted by asterisks. Figure 3: Effect of AmiA Wch derivatives on lysis of Caulobacter crescentus . ( a ) Overnight cultures of C. crescentus harbouring different constructs were left static at 30 °C and OD 600 nm were recorded every 90 min. Lysis occurred in strains carrying [P van −amiA Wch ] and [P van −( amiA-nlpD ) Wch ] while OD 600 nm of strains carrying [P van −amiA Wch H124A ], [P van −amiA Wch H55A E70A H124A E194A ], [P van −nlpD Wch ] and pMT335 were not affected. Error bars show the s.d. Data are from three biological replicates. ( b ) Muropeptide analysis of Caulobacter crescentus cell walls in the indicated strains harbouring different constructs as indicated on the figure. Differences among HPLC profiles are highlighted by asterisks. Full size image As E. coli amidase mutants have compromised LPS-dependent outer membrane barrier function, they are unable to grow on medium containing detergents, including the bile acid deoxycholate in McConkey agar [18] , [25] ( Fig. 2b ). Moreover, LPS is the receptor for bacteriophage ϕP1 and the Δ ABC mutant displays an increased resistance towards ϕP1 compared with WT cells ( Fig. 2c ). Surprisingly, expression of WT AmiA Wch corrected these deficiencies as well, while the AmiA Wch catalytic mutants were unable or substantially reduced in their ability to support these functions ( Fig. 2b,c ). The Δ ABC mutant is also sensitive to exogenously applied lysozyme (a muramidase) or bacitracin (an antibiotic interfering with C55~\nP recycling through inhibition of the kinase BacA; Figs 1b and 2d,e ). While expression of AmiA Eco corrects all deficiencies of the Δ ABC mutant ( Fig. 2a–f ), AmiA Wch was unable to correct the bacitracin sensitivity of the Δ ABC mutant. We attribute this to the ectopic (lytic) activity of AmiA Wch that, in the absence of the autoinhibitory region that is found in amidases such as AmiA Eco ( Supplementary Fig. 1 ), leads to ‘ghost’ cell formation and an imbalance in PG precursors and/or bactoprenol (C55~\nP) derivatives. Such an imbalance in C55~\nP might sensitize cells to inhibitors of the bactoprenol recycling pathway such as bacitracin. Taken together, we conclude that despite the massive genome reduction during the evolution of Chlamydiae , the coding sequence of a functional and lytic amidase has been retained. To confirm that AmiA Wch is indeed expressed in dividing W. chondrophila cells, we measured the abundance of the amiA Wch transcripts by reverse transcription quantitative (RT)–PCR post-infection (p.i.) of Vero host cells infected with W. chondrophila ( Fig. 4a ). We also raised polyclonal antibodies to AmiA Wch and probed for the presence of AmiA Wch by immunoblotting during growth of W. chondrophila ( Supplementary Fig. 4 ). These experiments revealed the amiA Wch transcript and the AmiA Wch translation product to be detectable at all time points p.i. Moreover, we used the anti-AmiA Wch antiserum for immunofluorescence microscopy of cells 24 h p.i. and observed AmiA Wch in clusters in the cell envelope and occasionally at the septum in deeply constricted cells ( Fig. 4b ). While our functional and cytological analyses provide compelling evidence that the chlamydial amidases are functional, expressed and at the correct subcellular compartment to process a PG-like polymer (synthesized by the PBP transpeptidases, PBP2 and/or PBP3) [5] , [6] , we cannot rule out that AmiA Wch acts directly on the PG building block lipid II, splicing off the MurNAc-GlcNAc disaccharide once lipid II is flipped onto the periplasmic face of the cytoplasmic membrane and polymerized by PBPs ( Fig. 1b ). In fact, the companion paper by Klöckner et al. [26] demonstrates that Chlamydiae pneumoniae AmiA can cleave lipid II in vitro . We thus hypothesize that AmiA is constitutively active and can release the MurNAc-GlcNAc disaccharide unit from Lipid II and/or from a septal/peripheral PG-like polymer, even in the absence of a topological amidase activator [3] , [4] , [22] . It is also conceivable that chlamydial AmiA orthologs are important for bactoprenol (C55~\nP) recycling, which could be limiting due to ongoing LPS (O-antigen) precursor biosynthesis as in E. coli [17] ( Fig. 1a ). 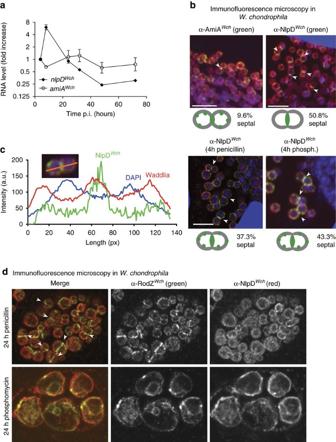Figure 4: NlpDWchlocalizes to the chlamydial division septum. (a) Transcript levels ofamiAWchandnlpDWchin Vero cells at different time points p.i. withW. chondrophila. Error bars show the s.d. Data are from three biological replicates. (b) NlpDWchlocalizes at the division plane (middle), while AmiAWchis localized at cell periphery with accumulation at constriction in dividing bacteria. Septal localization of NlpDWchis not affected by 4 h of penicillin or phosphomycin (phosph.) treatment (500 μg ml−1) administered 2 h p.i. Numbers indicate the fraction of cells with septal signal (n=100). Shown are merged images of cells stained with DAPI (blue), anti-Waddliaantibodies (red) and antibodies (green) to either AmiAWch(α-AmiAWch) or NlpDWch(α-NlpDWch). (c) Enrichment of NlpDWchat the division plane is not due to overlapping cells. Z-stacks were observed by confocal immunofluorescence microscopy. Reconstruction of a vertical cut through the cells is depicted here (inset). Quantification of pixel (px) intensities using ImageJ confirmed a concentration of NlpDWchat the division plane (right). (d) Immunofluorescence micrographs using antibodies to NlpDWch(red) and RodZWch(green) showing the delocalization of NlpDWchafter 24 h of penicillin and phosphomycin administered 2 h p.i. Note that the midcell localization of RodZWchis maintained in the presence of penicillin, but not in the presence of phosphomycin as published previously11. Figure 4: NlpD Wch localizes to the chlamydial division septum. ( a ) Transcript levels of amiA Wch and nlpD Wch in Vero cells at different time points p.i. with W. chondrophila . Error bars show the s.d. Data are from three biological replicates. ( b ) NlpD Wch localizes at the division plane (middle), while AmiA Wch is localized at cell periphery with accumulation at constriction in dividing bacteria. Septal localization of NlpD Wch is not affected by 4 h of penicillin or phosphomycin (phosph.) treatment (500 μg ml −1 ) administered 2 h p.i. Numbers indicate the fraction of cells with septal signal ( n =100). Shown are merged images of cells stained with DAPI (blue), anti- Waddlia antibodies (red) and antibodies (green) to either AmiA Wch (α-AmiA Wch ) or NlpD Wch (α-NlpD Wch ). ( c ) Enrichment of NlpD Wch at the division plane is not due to overlapping cells. Z-stacks were observed by confocal immunofluorescence microscopy. Reconstruction of a vertical cut through the cells is depicted here (inset). Quantification of pixel (px) intensities using ImageJ confirmed a concentration of NlpD Wch at the division plane (right). ( d ) Immunofluorescence micrographs using antibodies to NlpD Wch (red) and RodZ Wch (green) showing the delocalization of NlpD Wch after 24 h of penicillin and phosphomycin administered 2 h p.i. Note that the midcell localization of RodZ Wch is maintained in the presence of penicillin, but not in the presence of phosphomycin as published previously [11] . Full size image Amidases and endopeptidases influence LPS barrier function Since E. coli amidases are required for proper LPS-dependent barrier function, they could modulate signalling by Toll-like innate immune receptors that detect bacterial cell envelope components such as LPS. To investigate how AmiA Wch promotes LPS-dependent barrier function in E. coli Δ ABC cells, we isolated a spontaneous Δ ABC suppressor mutant (Δ ABC nlpI W24STOP ) that is able to grow on McConkey agar (supplemented with 0.5% Glucose; Fig. 5a ). While this mutant exhibits near WT sensitivity to ϕP1 ( Fig. 2c ), the defects in cell separation, lysozyme and bacitracin sensitivity were not mitigated ( Figs 2c,d and 5b ). Thus, the LPS-dependent barrier function can be genetically uncoupled from cell separation. 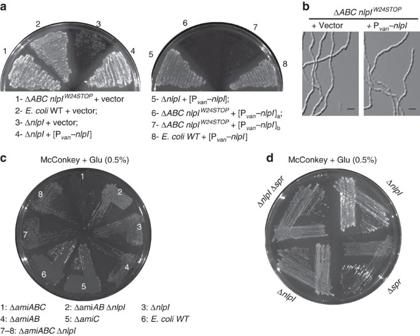Figure 5: Amidase and endopeptidase control LPS-dependent barrier function inE. coli. (a) Effect ofnlpIloss on growth on McConkey agar supplemented with 0.5% glucose (McCG) inWTand ΔABCstrains. NlpI expression in ΔABC nlpIW24STOPprevents growth on McCG. Note that the presence of the vector appears to compromise growth of thenlpImutant. (b) Representative DIC micrographs of ΔABCnlpIW24STOPharbouring the empty vector and a derivative carryingnlpI. Scale bar, 4 μm. (c)nlpI-dependent effect on McCG growth in different amidases mutant backgrounds, relative toWTand ΔABC. Deletion ofnlpIin the ΔABCmutant restores the ability to grow on McCG on the indicated strains. (d) Deletion ofnlpIin Δsprcells restores the ability to grow on McCG agar plates on the indicated strains. Figure 5: Amidase and endopeptidase control LPS-dependent barrier function in E. coli . ( a ) Effect of nlpI loss on growth on McConkey agar supplemented with 0.5% glucose (McCG) in WT and Δ ABC strains. NlpI expression in Δ ABC nlpI W24STOP prevents growth on McCG. Note that the presence of the vector appears to compromise growth of the nlpI mutant. ( b ) Representative DIC micrographs of Δ ABCnlpI W24STOP harbouring the empty vector and a derivative carrying nlpI . Scale bar, 4 μm. ( c ) nlpI -dependent effect on McCG growth in different amidases mutant backgrounds, relative to WT and Δ ABC . Deletion of nlpI in the Δ ABC mutant restores the ability to grow on McCG on the indicated strains. ( d ) Deletion of nlpI in Δ spr cells restores the ability to grow on McCG agar plates on the indicated strains. Full size image Genome re-sequencing of this suppressor mutant disclosed a nonsense mutation of the tryptophan codon at position 24 (TGG→TAG) in the nlpI gene, encoding a t etratrico p eptide r epeat (TPR)-containing lipoprotein required for virulence and adhesion in neonatal meningitis E. coli [27] , [28] . In support of the notion that the nlpI W24STOP mutation is a loss-of-function allele, expression of WT nlpI from a plasmid in the Δ ABC nlpI W24STOP quadruple mutant again conferred the growth defect on McConkey agar medium typical of Δ ABC cells ( Fig. 5a ). Conversely, deletion of nlpI (Δ nlpI :: cm R ) from Δ ABC cells enabled growth of the resulting Δ ABC Δ nlpI quadruple mutant on McConkey agar ( Fig. 5c ). How might NlpI act? Since Δ ABC nlpI W24STOP quadruple mutant cells are nearly as sensitive to bacitracin compared with the Δ ABC parent, it is unlikely that NlpI acts in the bactoprenol (C55~\nP) recycling pathway ( Fig. 1b ). Interestingly, nlpI is known to interact genetically with spr , a gene encoding a DD-endopeptidase that cleaves the peptide cross-bridges between m-DAP and D -alanine in PG [29] . Moreover, loss-of-function mutations in nlpI or overproduction of the m-DAP- D -alanine DD-endopeptidase Pbp7 both suppress the conditional lethality of an spr deletion (Δ spr ) mutant [30] , [31] . Consistent with the notion that inactivation of nlpI affects and perhaps loosens septal PG, we observed that the poor growth of a Δ spr strain on McConkey agar is attenuated by a Δ nlpI mutation ( Fig. 5d ), that Δ nlpI cells are sensitive towards increased expression of Spr or its paralogue YdhO ( Fig. 6a ) and that the inactivation of nlpI in WT or Δ ABC cells resulted in an increased muro-tetrapeptide monomer to dimer ratio as determined by HPLC analysis ( Table 1 ; Supplementary Fig. 5A,B ). On the basis of these results, we propose that NlpI (perhaps via the TPR repeat) negatively regulates Spr and other endopeptidases that convert muro-tetrapeptide dimers to monomers. Thus, a proper balance of amidase and DD-endopeptidase activities governs the barrier function of LPS. 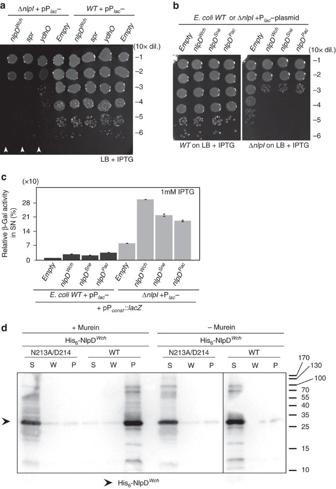Figure 6: Phenotypic and biochemical characterization of NlpDWch. (a) Effect of overexpression of NlpDWchfrom pTrc99a (vector) phenocopies the effect of Spr and YdhO overproduction on plating efficiency ofE. coli WTand ΔnlpIcells. Shown is a dilution series of the indicated strains. (b) Effect of overexpression of NlpDWch, NlpDSneor NlpDPacfrom Placon pSRK on plating efficiency ofWTand ΔnlpI E. colicells. Shown is a dilution series of cells carrying pSRK (vector) derivatives expressing NlpDWchfrom Placplated on LB with or without inducer (1 mM IPTG) of the indicated strains. (c) Lytic activity of NlpDWch, NlpDSneor NlpDPacexpressed from Placon pSRK inWTand ΔnlpI E. colicells carrying the LacZ-expressing plasmid pLac290-Pconst::lacZ(used because theE. coliparent, TB28, islacZminus). Beta-galactosidase activities were measured on SN of induced and non-induced cultures ofWT E. colicarrying Plac-nlpDconstructs. Error bars show the s.d. Data are from three biological replicates. (d) Binding of different His6-NlpDWchvariants toE. colimurein (PG) sacculi. PurifiedWTand mutant NlpDWch(3 μg each) were incubated with or without 1 mg ofE. colisacculi. Sacculi were pelleted by ultracentrifugation and washed once with buffer. Immunoblotting with antibodies to NlpDWchwas used to reveal NlpDWchin the supernatant (S), the wash fraction (W) or the pellet (P) fraction. The size markers (in kDa) are indicated on the right. The arrow on the left denotes the position of His6-NlpDWch. Figure 6: Phenotypic and biochemical characterization of NlpD Wch . ( a ) Effect of overexpression of NlpD Wch from pTrc99a (vector) phenocopies the effect of Spr and YdhO overproduction on plating efficiency of E. coli WT and Δ nlpI cells. Shown is a dilution series of the indicated strains. ( b ) Effect of overexpression of NlpD Wch , NlpD Sne or NlpD Pac from P lac on pSRK on plating efficiency of WT and Δ nlpI E. coli cells. Shown is a dilution series of cells carrying pSRK (vector) derivatives expressing NlpD Wch from P lac plated on LB with or without inducer (1 mM IPTG) of the indicated strains. ( c ) Lytic activity of NlpD Wch , NlpD Sne or NlpD Pac expressed from P lac on pSRK in WT and Δ nlpI E. coli cells carrying the LacZ-expressing plasmid pLac290-P const ::lacZ (used because the E. coli parent, TB28, is lacZ minus). Beta-galactosidase activities were measured on SN of induced and non-induced cultures of WT E. coli carrying P l ac - nlpD constructs. Error bars show the s.d. Data are from three biological replicates. ( d ) Binding of different His 6 -NlpD Wch variants to E. coli murein (PG) sacculi. Purified WT and mutant NlpD Wch (3 μg each) were incubated with or without 1 mg of E. coli sacculi. Sacculi were pelleted by ultracentrifugation and washed once with buffer. Immunoblotting with antibodies to NlpD Wch was used to reveal NlpD Wch in the supernatant (S), the wash fraction (W) or the pellet (P) fraction. The size markers (in kDa) are indicated on the right. The arrow on the left denotes the position of His 6 -NlpD Wch . Full size image Table 1 Changes in muropeptides in various E. coli strains. Full size table Septal localization and cell wall remodelling by NlpD Wch Prompted by these functional interactions between the amidases and DD-endopeptidases in E. coli , we searched for putative DD-endopeptidases encoded in the W. chondrophila genome using E. coli Spr, YdhO and YebA as BLASTP queries. After considering the genomic context where the candidates are encoded, we focused our attention on the gene annotated as nlpD ( nlpD Wch ). nlpD Wch is embedded within a cluster of genes predicted to code for cell wall and division functions ( Fig. 1c ). Although it is difficult to predict from the primary structure if the NlpD Wch translation product has endopeptidase activity, the presence of two putative LysM domains ( Fig. 1d ; Supplementary Fig. 6 ) that are known to mediate PG-binding and/or septal localization in other proteins [32] along with a 36% similarity with NlpD Eco ( Supplementary Fig. 6 ) make it a strong candidate to act in remodelling of a PG-like polymer and/or chlamydial division. Having shown that the E. coli Δ nlpI :: cm R cells are a suitable background in which to probe for endopeptidase activity, we then tested whether expression of NlpD Wch reduces the plating efficiency of Δ nlpI :: cm R cells, akin to expression of Spr or YdhO, without affecting WT cells ( Fig. 6a ). Indeed, WT NlpD Wch but not mutant variants harbouring missense mutations in conserved residues within the LysM domain ( Supplementary Fig. 6 ) caused a strong reduction in plating efficiency of Δ nlpI :: cm R cells compared with WT cells ( Supplementary Fig. 7A ). Several of these missense mutants accumulated NlpD Wch to similar levels as WT ( Supplementary Fig. 7B ), suggesting that conserved residues in the LysM domain are required for function. A similar reduction in plating efficiency was observed upon expression of the NlpD orthologue from Simkania negevensis or Parachlamydia acanthamoebae (NlpD Sne or NlpD Pac , respectively) in Δ nlpI :: cm R cells, but not in WT E. coli ( Fig. 6b ). Moreover, induction of NlpD Wch , NlpD Sne or NlpD Pac expression caused an efficient release of LacZ from E. coli Δ nlpI :: cm R cells and only poorly from WT E. coli cells ( Fig. 6c ). To confirm that NlpD Wch can affect E. coli PG, we conducted HPLC analysis of muropeptides released from sacculi of Δ ABC cells expressing NlpD Wch . This revealed a similar increase in muro-tetrapeptide monomer to dimer ratio ( Table 1 ; Supplementary Fig. 5A,B ) compared with the empty vector, as that resulting from the loss of NlpI. Interestingly, the increase in tetrapeptide monomer to dimer ratio was mitigated upon co-expression of AmiA Wch with NlpD Wch ( Table 1 ; Supplementary Fig. 5 ), despite near-identical steady-state levels of NlpD Wch in cells with the AmiA Wch -NlpD Wch co-expression compared with cells with the NlpD Wch single expression plasmid ( Supplementary Fig. 2C ), suggesting that AmiA Wch is epistatic over NlpD Wch and, thus, that they act in the same pathway. Next, we explored the expression and localization of NlpD Wch in W. chondrophila grown in Vero cells. RT–PCR ( Fig. 4a ) and immunoblotting using polyclonal antibodies to NlpD Wch ( Supplementary Fig. 4 ) showed that NlpD Wch is indeed expressed. Importantly, IFM performed on Vero cells 24 h p.i. with W . chondrophila revealed fluorescent bands of NlpD Wch at midcell in 50.8±1.1% of constricted cells ( Fig. 4b ) and it can already be seen at the septum early during constriction (in 47% of the cells, Supplementary Fig. 8 ), with a significant increase in frequency at the later stages of constriction. Quantitative analysis of the fluorescence traces from NlpD Wch , DAPI (4′,6-diamidino-2-phenylindole)-stained chromosome and the anti- Waddlia -stained cell envelope revealed a sharp increase in NlpD Wch abundance at the medial site, in between two broad peaks of DAPI-stained DNA flanked by the cell envelope ( Fig. 4c ). This septal localization is still maintained for 4 hours after inhibition of division with penicillin, an inhibitor of PG transpeptidation enzymes (Pbp2/3), or with phosphomycin, an inhibitor of the lipid II biosynthetic enzyme MurA ( Fig. 4b ). However, 20 h later only peripheral NlpD Wch was observed under both conditions (septal only in 4.4% and 2.4% of dividing cells, respectively; Fig. 4d and Supplementary Fig. 8 ). By contrast, the early cell division marker RodZ Wch was still septal in the presence of the transpeptidation inhibitor (septal in 43.4% of dividing cells), but not when lipid II biosynthesis is blocked ( Fig. 4d ), as reported recently [11] . As these findings suggest that chlamydial NlpD is recruited to the division septum by its substrate, a PG-like D-amino acid-containing peptide polymer, we used a pelleting assay with intact and purified E. coli polymeric PG (sacculi) to determine whether purified WT or mutant His 6 -tagged NlpD Wch (His 6 -NlpD Wch ) can indeed bind polymeric PG in vitro ( Fig. 6d ). E. coli sacculi pulled down WT His 6 -NlpD Wch , but not mutant derivative lacking two conserved residues in the LysM domain (N213A/D214A; Supplementary Fig. 6 ), indicating that NlpD Wch can bind PG directly. Our data support a model in which NlpD Wch recognizes a PG-like polymer at the division septum, while AmiA trims this polymer or lipid II molecules throughout the envelope and possibly at the division furrow in the final stages of division, perhaps to lower NOD1/2-inducing MurNAc-peptide signals [12] , [33] during chlamydial infections, akin to the staphylococcal autolysins that prevent detection by the Drosophila innate immune system [33] . Interestingly, a PG-like polymer was recently extracted from the ‘environmental’ chlamydia Protochlamydia amoebophila , an amoebal symbiont, but similar attempts were unsuccessful for Simkania negevensis [34] . Nevertheless, we found that the S. negevensis genome encodes functional AmiA and NlpD (AmiA Sne and NlpD Sne ) that are active on E. coli PG, suggesting that PG-like material is also present in S. negevensis. It is possible that pervasive PG synthesis throughout the envelope (giving rise to intact sacculi) is a feature of chlamydial lineages that establish symbiotic relationships with amoebae, while chlamydial human pathogens only produce a cryptic, modified, short-lived, thin and/or spatially restricted PG. In light of the recent evidence that PG synthesis can indeed occur de novo (that is, in the absence of a preexisting template) in Bacillus subtilis cells [35] , it is conceivable that a PG-like structure is confined temporally and spatially to the division septum in chlamydial pathogens. Recent experiments using fluorescently labelled D -amino-dipeptides provided evidence of a septal peptide component in PG (or in lipid II) of Chlamydia trachomatis [10] , in support of the earlier discovery of the SEP antigen (recognized by antibodies raised against the mycobacterial cell wall containing RIBI adjuvant) at the division septum of C. trachomatis and Chlamydia psittaci [9] . Our data indicate that a septal PG-like polymer in the human chlamydial pathogen W. chondrophila is both a substrate and an important localization cue for a septal PG-binding protein (NlpD) during chlamydial cell division. Moreover, using purified components Klöckner et al. [26] provide compelling biochemical evidence that C. pneumoniae NlpD has carboxypeptidase activity in vitro . The notion that human chlamydial pathogens rely on a PG-like peptide polymer at the division site and that they localize NlpD to this site in the absence of an FtsZ homologue raises the important evolutionary question how a PG-like division septum is positioned in different bacteria. Our recent identification of the RodZ homologue RodZ Wch as an early septal protein [11] along with the finding reported here that RodZ Wch is still septal under conditions when NlpD Wch is dispersed (in the presence of penicillin) suggest that RodZ Wch localizes to the septum before NlpD Wch and that it could play a key role in orchestrating septal assembly (via PBPs) and dissolution (via NlpD Wch and possibly AmiA Wch ). While FtsZ is known to be dispensable in another bacterial phylum (the Firmicutes) when PG is absent [13] , [14] , the only known case of FtsZ-independent PG-based septation has been described for filamentous bacteria from the phylum Actinobacteria (genus Streptomyces ) that rely on FtsZ exclusively for septation during spore development, while crosswalls formed during vegetative (hyphal) growth do not require FtsZ [36] . As the Streptomyces do not encode an obvious RodZ orthologue in their genomes, different solutions have emerged for the synthesis of a PG-based septum and the subsequent recruitment of remodelling enzymes in diverse bacterial phyla and even in eukaryotic organelles [1] , [37] . Bacterial strains and growth conditions Strains and plasmids used in this study are listed in Supplementary Table 2 and their constructions are described in the Supplementary Methods section. E. coli strains were grown at 30 °C in Luria–Bertani (LB) broth, LB-agar [38] or McConkey agar supplemented with gentamycin (10 μg ml −1 ), IPTG (isopropyl-β-thio-galactopiranoside, 1 mM), as needed or otherwise indicated. C. crescentus strains were grown at 30 °C in peptone yeast extract supplemented with gentamycin (1 μg ml −1 ) as needed. Plasmids were introduced in E. coli by electroporation, chemical transformation or conjugation. W. chondrophila ATCC VR-1470 T was grown in Vero cells as previously described [5] . Overnight cell cultures containing originally 10 5 cells ml −1 were infected with a 2,000 × dilution of W. chondrophila . The cells were then centrifuged for 15 min (to improve contact of W. chondrophila ) at 1,790 g , incubated 15 min at 37 °C and washed with PBS before addition of fresh media. Differential interference contrast microscopy Cultures were grown at 30 °C in LB medium unless otherwise indicated. Unless otherwise indicated cells were imaged by DIC (Differential Interference Contrast) optics on microscope slides harbouring a thin (1%) agarose pad. A Zeiss Axioplan 2 microscope fitted with an HQ Snapshot camera, a Zeiss oil immersion objective ( × 100/1.45 numerical aperture) were used to acquire DIC images using software from Metamorph (Universal Imaging). Cells and ghosts were quantified using ImageJ software ( http://rsbweb.nih.gov/ij/ ). Immunofluorescence and confocal microscopy Infected Vero cells on coverslips were fixed with ice-cold methanol for 5 min at room temperature. Infection rate, inclusions and aberrant bodies were quantified by fluorescence microscopy by counting a minimum of hundred cells in duplicate [5] . Images were taken by confocal microscopy using a Zeiss LSM 510 Meta (Zeiss, Oberkochen, Germany). Images were then treated and quantified using ImageJ software. AmiA and NlpD purification and production of antibodies His 6 -NlpD Wch protein and the N213A/D214A mutant derivative were expressed from pET28a in E. coli Rosetta (DE3)/pLysS (Novagen, Madison, WI) and purified under native conditions using Ni 2+ chelate chromatography. A 5 ml overnight culture was diluted into 1 l of pre-warmed LB. OD 600 nm were monitored until OD 600 nm =~\n0.3–0.4, then 1 mM IPTG was added to the culture and growth continued. After 3 h cells were pelleted, and resuspended in 25 ml of lysis buffer (10 mM Tris HCl (pH 8), 0.1 M NaCl, 1.0 mM β-mercaptoethanol, 5% glycerol, 0.5 mM imidazole Triton X-100 0.02%). Cells were sonicated (Sonifier Cell Disruptor B - 30 ; Branson Sonic Power. Co., Danbury, CT) on ice using 12 bursts of 20 s at output level 5.5. After centrifugation at 4,300 g for 20 min, the supernatant was loaded onto a column containing 5 ml of Ni-NTA agarose resin pre-equilibrated with lysis buffer. Column was rinsed with lysis buffer, 400 mM NaCl and 10 mM imidazole, both prepared in lysis buffer. Fractions were collected (in 300 mM Imidazole buffer, prepared in lysis buffer) and used to immunize New Zealand white rabbits (Josman LLC, Napa, CA). His 6 -SUMO-AmiA Wch was expressed from pCWR547- amiA Wch over in E. coli Rosetta (DE3)/pLysS and purified in denaturing buffer (8 M Urea, 100 mM NaH 2 PO 4 , 25 mM Tris). A 5 ml overnight culture was diluted into 1L of pre-warmed LB. OD 600 nm was monitored until OD 600 nm =~\n0.3–0.4, then 1 mM IPTG was added to the culture transferred at room temperature for 5 h. Thereafter, cells were pelleted, resuspended in 25 ml of lysis buffer (10 mM Tris HCl (pH 8), 0.1 M NaCl, 1.0 mM β-mercaptoethanol, 5% glycerol, 0.5 mM imidazole, Triton X-100 0.02%). Cells were sonicated (Sonifier Cell Disruptor B - 30 ; Branson Sonic Power. Co., Danbury, CT) on ice using 12 bursts of 20 s at output level 5.5. After centrifugation at 4,300 g for 20 min, the supernatant were discarded and the pellet resuspended in 25 ml of Buffer B (denaturing buffer, pH 8.0), then centrifuged at 4,300 g for 20 min, the supernatant was loaded onto a column containing 5 ml of Ni-NTA agarose resin. Column was rinsed with Buffer B, Buffer C (denaturing buffer, pH 6.3) and eluted with Buffer E (denaturing buffer, pH 4.5). Fractions were collected, the protein was excised from a 15% SDS polyacrylamide gel and used to immunize New Zealand white rabbits (Josman LLC, Napa, CA). Immunoblots Pelleted cells were resuspended in 1 × SDS sample buffer (50 mM Tris–HCl (pH 6.8), 2% SDS, 10% glycerol, 1% β-mercaptoethanol, 12.5 mM EDTA, 0.02% Bromophenol Blue), heated to 95 °C for 10 min and stored at −20 °C. The resulting cell extracts were resolved on SDS–PAGE gels and transferred onto PVDF (polyvinylidenfluoride) membranes. PVDF membranes (Merck Millipore Headquarters, Billerica, MA) were blocked with TBS, 0.05% Tween 20 and 5% dry milk for 1 h and then incubated for 1 h with the primary antibodies diluted in TBS, 0.05% Tween 20 and 5% dry milk. The different antisera (custom produced, as described above) were used at the following dilutions: anti-AmiA Wch (1:10,000), anti-NlpD Wch (1:10,000). The membranes were washed four times for 5 min in TBS and incubated 1 h with the secondary antibody (HRP-anti-Rabbit 1:10,000) diluted in TBS, 0.05% Tween 20 and 5% dry milk. The membranes were finally washed again four times for 5 min in TBS and revealed with Immobilon Western Blotting Chemoluminescence HRP substrate (Merck Millipore Headquarters, Billerica, MA). Phage manipulation, lysozyme and antibiotic sensitivity tests The bacterial strains used in the present study were used to produce ΦP1 lysates and tested for phage P1 sensitivity [38] . Saturated cultures of E. coli TB28 (Δ lacZYA<>frt ) were used to produce ΦP1 lysates. Cells from overnight cultures were diluted 1:100 in LB with 25 mM CaCl 2 and infected with ΦP1 lysate. Phage titres were calculated by spot and plating methods. Briefly 1.5 ml of cells from overnight cultures were pelleted and resuspended in 0.3 ml of LB with 5 mM of CaCl 2 , and then incubated for 10 min at 37 °C. A total of 0.05 ml of ΦP1 were added to the suspension and incubated at 37 °C for 20 min. Serial dilution of the suspension were made and added to 4 ml of LB top agar supplemented with 5 mM CaCl 2 , plates were then incubated overnight at 37 °C or until plaques are visible. The titre of the phage was calculated as plaque-forming units (pfu) per ml, then percentage of the titre relative to WT E. coli was calculated and reported as the log 10 of the percentage. Values reported in the figures come from three independent biological replicas. Sensitivity of bacterial strains presented in this study were determined as follows: 5 mg of lysozyme (AppliChem) and bacitracin (Sigma), respectively, were spotted on LB top agar containing 0.250 ml of saturated overnight cultures of the strains to be tested and incubated overnight at 30 °C. Diameter of the inhibition halo was measured from three biological replicates. Muropeptide analysis Chemical composition of PG was determined by the standardized procedure developed by Cecolabs (Tübingen, Germany). For PG isolation and characterization the strains were grown overnight in LB or peptone yeast extract media unless otherwise indicated. Cells were harvested by centrifugation (4,300 g , 20 min at 4 °C), supernatant was discarded and cells resuspended in 20 ml of phosphate buffered saline (pH 7.4; 1x PBS) and then boiled for 15 min, the resulting extract was centrifuged and after discarding the supernatant the pellet was stored at 4 °C. Briefly, cell pellets were resuspended and boiled in SDS, cell wall material was harvested by centrifugation and broken with glass beads. Broken cell wall was digested with mutanolysin and analysed by HPLC [39] . HPLC analyses were performed with an Agilent 1200 system with a Prontosil C18-RP column (Bischoff Chromatography, Leonberg, Germany) [40] . Selected peaks were identified by matrix-assisted laser desorption ionization and electrospray mass spectrometry. Quantitative analysis of selected peaks was done by integration of the peak area using the trapezoidal rule. The area of each peak was then used to derive the ratios of cell wall components among the different strains. Murein (sacculi) pull-down assay NlpD Wch -His 6 and NlpD Wch N213A D214A -His 6 were overproduced in E. coli Rosetta (λDE3)/pLys. Proteins were purified by nickel affinity chromatography as described above, concentrated by ultrafiltration in Amicon 3K columns (Millipore) and stored at −80 °C in Binding buffer (20 mM Tris–HCl, 1 mM MgCl 2 30 mM NaCl, 0.05% Triton X-100, pH 6.8) containing 50% glycerol. Bradford assay was used to determine the protein concentration in each sample. E. coli murein (sacculi) was purchased from Cecolabs (Tuebingen, Germany) and resuspended in binding buffer at a concentration of 10 mg ml −1 . Proteins (3 μg or 6 μg) were added to 1 mg murein in a total volume of 100 μl and incubated on ice for 30 min. Murein from samples was collected by centrifugation in a Beckman SW55Ti rotor at 303,648 g for 30 min at 4 °C. Sedimented murein was resuspended in 0.1 ml of cold binding buffer and centrifuged again. Murein pellets were resupended in 0.02 ml of cold binding buffer. The supernatant of the first centrifugation step (S), the supernatant of the washing step (W) and the pellet (P) were analysed by SDS–PAGE followed by immunoblot with anti-NlpD antiserum (see immunoblots for details). Assay to determine the lytic activity of chlamydial amidases WT and Δ ABC E. coli cells harbouring pSRK (P lac− ) and pMT335 (P van− ) amidase plasmids were transformed with the low copy plasmid pLac290 harbouring a promoter of C. crescentus , which is constitutively active in E. coli (pLac290-P const ::lacZ ). Overnight cultures were diluted in fresh LB and incubated at 30 °C for 6 h. Culture supernatants (SN) were collected by centrifugation at 20,000 g for 5 min at room temperature. SN were diluted 1:10 in 1 ml of LB and 0.2 ml of diluted SN were used for standard β-Galactosidase (LacZ) assay [38] . Quantitative real-time PCR Infection of Vero cells by W. chondrophila was quantified by quantitative PCR [11] . At different time points after infection, infected cells were resuspended by scratching. Genomic DNA was extracted from 50 μl of cell suspension using the Wizard SV Genomic DNA purification system (Promega, Madison, WI). Elution was processed with 200 μl of water. Quantitative PCR was performed using iTaq supermix with ROX (BioRad, Hercules, CA). To detect W. chondrophila , 200 nM of primers WadF4 and WadR4, 100 nM of probe WadS2 and 5 μl of DNA were used. Cycling conditions were 3 min at 95 °C followed by 40 cycles of 15 s at 95 °C and 1 min at 60 °C for both PCRs. A StepOne Plus Real-time PCR System (Applied Biosystems, Carlsbad, CA) was used for amplification and detection of the PCR products. How to cite this article: Frandi, A. et al. FtsZ-independent septal recruitment and function of cell wall remodelling enzymes in chlamydial pathogens. Nat. Commun. 5:4200 doi: 10.1038/ncomms5200 (2014).